Maximizing single-pass conversion does not result in practical readiness for CO2reduction electrolyzers 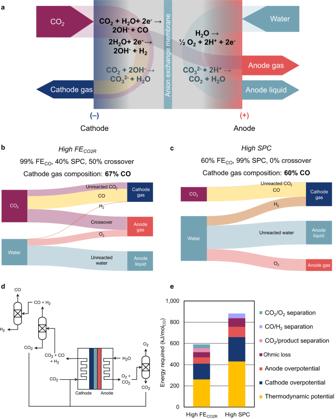Fig. 1: Typical CO2electrolyzer outlet gases. aReaction pathways for a typical CO2electrolyzer reducing CO2to CO in a neutral electrolyte with an anion exchange membrane. Black text indicates heterogeneous redox reactions, while blue indicates homogeneous reactions.b,cMolar flow rates in a single pass of CO2reduction to CO for example scenarios with (b) high Faradaic efficiency towards CO2R with realistic parameters and (c) high single-pass conversion with optimistic parameters. The total current is the same in both cases. Despite optimistically high single-pass conversion in (c), CO concentration in the cathode outlet is decreased.dSample gas separation scheme required for a CO2electrolyzer.eEnergy required per mole of product for reaction (modeled as overpotential) versus separation (modeled thermodynamically) shows that the high-SPC scenario wastes reactor energy on hydrogen evolution. Process parameters correspond to (b) and (c). 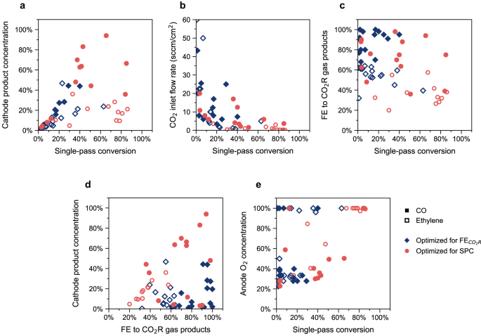Fig. 2: Correlations between single-pass conversion and CO2R performance in literature. aHigh single-pass conversion does not result in highly concentrated products that are suitable for downstream applications.bHigh single-pass conversion has been achieved at low feed flow rates, at which hydrogen evolution is the dominant reaction.cFaradaic efficiency to CO2R trades off with single-pass conversion across various reaction conditions.dConcentrated cathode streams are produced by maximizing Faradaic efficiency, which is extremely challenging at high single-pass conversions.eAnode gas separations can be minimized across a range of single-pass conversion. Hollow symbols () correspond to ethylene production and filled symbols () represent CO generation. Red circles () correspond to the highest single-pass conversion in a report, and blue diamonds () correspond to the highest FECO2Rin a report; their operating conditions are usually different since selectivity and SPC trade off in current electrolyzer configurations10,16,18,19,20,22,27,29,30,31,32,33,34,35,36,37,38,39,40,41,42,43,44,45,46,47,48,49. Outlet streams from CO 2 electrolyzers need gas separations Electrochemical CO 2 reduction is a potential low-carbon pathway for producing chemical feedstocks and fuels from renewable electricity, water, and CO 2 [1] , [2] . CO 2 electrolyzers can produce value-added chemicals whose industrial demand is in the hundreds of megatons annually [3] , [4] , including carbon monoxide [5] , formic acid [6] , and ethylene [7] . CO can in turn be electrochemically reduced in a two-stage cascade [8] , [9] . State-of-the-art CO 2 electrolyzers have limited reactant utilization because of the incomplete reaction of CO 2 , as well as CO 2 crossover due to carbonate acid-base equilibrium. Selectivity is also limited by competition from water reduction via the hydrogen evolution reaction (HER), in which CO 2 is uninvolved. Gas separations and recycle streams are needed to recover and convert unreacted CO 2 , and to purify products. Typical CO 2 electrolyzers produce two gas-phase outlet streams, one each at the cathode and anode, which can both contain residual CO 2 (Fig. 1a ). The cathode gas contains gas-phase CO 2 R products, unreacted CO 2 , and hydrogen as a byproduct from the HER. CO 2 electrolyzers can produce carbon monoxide with 100% molar selectivity [10] , [11] , so a hydrogen-free tail gas can be produced under optimal conditions. For multicarbon products, state-of-the-art electrolyzers have a molar selectivity of 50% to C 2+ products, with the co-evolution of 20% H 2 and 30% C 1 products at the cathode [12] , [13] . The scope of this discussion is limited to gas-phase separations, which are necessary for the production of CO or of ethylene, the dominant C 2+ product. For liquid products like formic acid, ethanol, and acetate, both gas and liquid product streams are formed, which requires an independent analysis of separations. Fig. 1: Typical CO 2 electrolyzer outlet gases. a Reaction pathways for a typical CO 2 electrolyzer reducing CO 2 to CO in a neutral electrolyte with an anion exchange membrane. Black text indicates heterogeneous redox reactions, while blue indicates homogeneous reactions. b , c Molar flow rates in a single pass of CO 2 reduction to CO for example scenarios with ( b ) high Faradaic efficiency towards CO 2 R with realistic parameters and ( c ) high single-pass conversion with optimistic parameters. The total current is the same in both cases. Despite optimistically high single-pass conversion in ( c ), CO concentration in the cathode outlet is decreased. d Sample gas separation scheme required for a CO 2 electrolyzer. e Energy required per mole of product for reaction (modeled as overpotential) versus separation (modeled thermodynamically) shows that the high-SPC scenario wastes reactor energy on hydrogen evolution. Process parameters correspond to ( b ) and ( c ). Full size image At the anode, oxygen is produced from water oxidation via the oxygen evolution reaction (OER). The anode outlet also contains CO 2 that crosses over the membrane via the homogeneous reactions shown in Fig. 1a [14] , [15] . This crossover arises from acid-base equilibria—hydroxide generated by the cathodic reaction converts dissolved CO 2 into (bi)carbonate ions in neutral electrolytes, like KHCO 3 or Cs 2 CO 3 , or alkaline electrolytes such as KOH. (Bi)carbonate anions migrate towards the anode, where they buffer protons generated by OER, regenerating CO 2 gas. This buffering reaction limits single-pass conversion at most pH [16] . In neutral electrolytes, carbonate ion crossover stoichiometrically consumes 0.5 mol CO 2 /mol e − , which results in an anode tail gas consisting of 67 mol% CO 2 + 33 mol% O 2 . Therefore, both the cathode and anode outlet gases can contain unreacted CO 2 that must be captured and recycled to the cathode (Fig. 1b, c ). Recycling unreacted CO 2 requires a gas separation that could be a capital- and energy-intensive process. An electrolyzer with incomplete conversion, imperfect selectivity, and reactant crossover needs at least three pairwise separations: one to separate the target product from byproducts, and two to recycle CO 2 from the cathode and anode outlets (Fig. 1d ). Separation units are typically modeled as pressure-swing adsorption using electrical utilities [3] , but cryogenic distillation or amine scrubbing could be preferable depending on process scale, stream compositions, and available utilities [17] . If extensive downstream separations are required to purify products and recycle CO 2 , the overall energy efficiency of CO 2 R has been argued to suffer unacceptably [15] . To account for separation demands, studies on CO 2 electrolyzers increasingly report single-pass conversion (SPC): 
    SPC=CO_2 moles converted to products/CO_2 moles fed to reactor
 In other catalytic processes, high SPC generally suggests improved reactant utilization and hence lower energy to recycle the unreacted feed. Also, downstream applications, like ethylene polymerization, typically require high-purity feedstocks. Since high SPC implies that the products are not diluted in leftover reactant, it is associated with marketable product streams. Molar stream composition is a critical consideration for downstream applications. For instance, thermal reactors are sensitive to reactant partial pressures, so CO 2 R products must often be concentrated for downstream processing. To assess the relationship between SPC and reactor outlet composition, we analyzed data from literature reports targeting state-of-the-art CO 2 electrolyzer performance (for details, see Supplementary Information , Section 3 ). These relationships are demonstrated in Fig. 2 , with additional representations in Fig. S2 and pH dependence in Fig. S3 . Fig. 2: Correlations between single-pass conversion and CO 2 R performance in literature. a High single-pass conversion does not result in highly concentrated products that are suitable for downstream applications. b High single-pass conversion has been achieved at low feed flow rates, at which hydrogen evolution is the dominant reaction. c Faradaic efficiency to CO 2 R trades off with single-pass conversion across various reaction conditions. d Concentrated cathode streams are produced by maximizing Faradaic efficiency, which is extremely challenging at high single-pass conversions. e Anode gas separations can be minimized across a range of single-pass conversion. Hollow symbols ( ) correspond to ethylene production and filled symbols ( ) represent CO generation. Red circles ( ) correspond to the highest single-pass conversion in a report, and blue diamonds ( ) correspond to the highest FE CO2R in a report; their operating conditions are usually different since selectivity and SPC trade off in current electrolyzer configurations [10] , [16] , [18] , [19] , [20] , [22] , [27] , [29] , [30] , [31] , [32] , [33] , [34] , [35] , [36] , [37] , [38] , [39] , [40] , [41] , [42] , [43] , [44] , [45] , [46] , [47] , [48] , [49] . Full size image As shown in Fig. 2a , we find that experimental conditions that maximize single-pass conversion do not correspond to concentrated product streams suitable for further reaction. To maximize SPC, studies are often conducted at low inlet CO 2 flow rates (Fig. 2b ). Under these conditions, the partial pressure of CO 2 drops steeply across the reactor as it is consumed by reaction, resulting in a loss in CO 2 R selectivity in favor of HER [18] , [19] , [20] . In some cases, SPC has also been increased using an acidic electrolyte (e.g. H 2 SO 4 + K 2 SO 4 ), or reverse-biased bipolar membrane to eliminate carbonate formation and crossover. Unfortunately, the high availability of protons in such configurations steers selectivity towards HER over CO 2 R, which is not captured in SPC since CO 2 plays no direct role in the HER reaction. This tradeoff between Faradaic efficiency (FE CO2R ) and SPC has been demonstrated for various electrolyzers previously [21] , [22] , [23] , and is reflected across the dataset we analyzed (Fig. 2c ). Hence strategies that reduce the need to recycle CO 2 still require separations to remove H 2 and concentrate the product for downstream processes. Additionally, electrolyzer energy is wasted on making H 2 in these scenarios. A comparison of the energy required for reaction and separation (Fig. 1e , Fig. S1 ) and a recent in-depth analysis [24] suggest that reactor energy requirements significantly exceed the energetic costs of separations. Hence the energy demand for CO 2 R is dramatically increased at high SPC/ low FE CO2R conditions, even if gas separations are reduced (Fig. 1e ). Therefore, high SPC neither eliminates the need for cathode gas separations, nor indicates that products are formed at an improved energy efficiency. Neither SPC nor FE CO2R directly reflect outlet composition, as indicated by the lack of a clear trend in Fig. 2a, d . While SPC fails to account for HER, FE CO2R and partial current density do not reflect molar flow rates. For C 2+ products, this problem is especially acute since multiple electron pairs are transferred for CO 2 R, compared to a single pair to make H 2 . For example, a 90% FE to CO with 10% to H 2 at 100% SPC translates to a stream composition of 90 mol% CO + 10 mol% H 2 . In contrast, 90% FE to ethylene with 10% to H 2 results in 60 mol% ethylene + 40 mol% H 2 because of the 12 e - transferred to produce ethylene. Although high FE CO2R does not perfectly scale to high molar flows, Fig. 2d shows that the most concentrated cathode product is obtained at high FE CO2R , which is extremely challenging to achieve at the low flow rates that give high SPC. At high current densities and FE CO2R , high crossover and selective reaction manifest in very concentrated cathode products. On the other extreme, crossover can be minimized to produce 100% O 2 at the anode. However, a pure O 2 anode stream has been reported across a range of SPC (Fig. 2e ), so high SPC is not a necessary condition for low crossover. If minimizing HER is important for CO 2 R scaleup, then SPC to CO 2 R products is a misleading metric that does not truly reflect that a reactor design is practical. To pursue industrial relevance for selective CO 2 R, we recommend a careful selection of metrics and operating conditions for measuring and reporting electrolyzer performance. Our analysis shows that SPC does not accurately reflect downstream compositions at the cathode. A realistic representation of separation demand can be provided by mole fractions and outlet flow rates. The concentration of products in the cathode and anode streams indicates the readiness of electrolyzers for downstream applications, informing separation energy and process feasibility. Therefore, we recommend that researchers report cathode and anode product stream compositions. Section 3 of the Supplementary Information outlines the conversions between more common metrics and stream compositions, which can also be used on existing datasets to analyze the effects of experimental variables on product streams. We suggest that researchers characterize the composition of the anode gas, as has been recommended by Seger and coworkers [25] , [26] . At present, very few reports on state-of-the-art CO 2 electrolyzers explicitly quantify the anode gas stream. The combination of complete anode and cathode gas quantification allows the carbon mass balance to be used as an additional experimental validation step. The carbon balance is especially important in alkaline electrolytes that absorb CO 2 , where anode gas quantification can be nuanced. CO 2 R reports in alkaline conditions rarely assess the extent of carbonate formation [27] or CO 2 regeneration at the anode, and often report a lower crossover than is physically reasonable. This may be due to the anolyte not being purged of CO 2 , thus excluding carbonate formation from the carbon balance. We recommend that researchers supply CO 2 flow rates that correspond to at least the amount of CO 2 consumed stoichiometrically by CO 2 R at the applied current. Many reports feed a lower CO 2 molar flow than the chronopotentiometry current. This artificially inflates SPC at the cost of selectivity, since the CO 2 R partial current density is severely reactant limited and HER must compensate for the remaining current. The complete reaction of 1 sccm of CO 2 accounts for 143 mA of current through a 2-e − pathway making C 1 products, or 430 mA of current through a 12-e − C 2 pathway. Therefore, on a 5 cm 2 cathode where 1 sccm CO 2 is fed, it is impossible to produce more than 29 mA/cm 2 of C 1 products, even in the absence of crossover. In a neutral electrolyte where carbonate is the dominant charge carrier, CO 2 R current is further constrained by the crossover of 0.5 mol CO 2 /mol e − . Under these conditions, the partial current density to 12-e − C 2+ products from 1 sccm CO 2 on a 5 cm 2 electrode is at most 22 mA/cm 2 . Most experiments in membrane electrode assemblies (MEAs) are operated at >50 mA/cm 2 , so low CO 2 flow rates guarantee high HER. To operate at a current density of 100 mA/cm 2 of CO 2 R to CO on a 5 cm 2 electrode in neutral conditions, at least 7 sccm of CO 2 must be fed to the reactor. From a scaleup perspective, the optimal flowrate depends on complex tradeoffs, including between electrolyzer energy and separator capital cost, or selectivity versus crossover [24] . CO 2 R has been shown to be severely limited by CO 2 availability in a variety of system configurations [10] , [20] , [28] . Continuum modeling of current electrolyzer designs suggests that concentration gradients on the cathode surface effectively make it impossible to co-optimize conversion and selectivity at low flow rates [28] . In contrast, large CO 2 feeds steer selectivity towards CO 2 R but increase separation and compression energies by diluting products and requiring recycle streams. Several reports [19] , [20] , [22] show a parabolic trend in product concentration versus feed flow rate. Further techno-economic analysis is needed to determine whether the process energy and cost are optimal at the peak of this parabola. We also note that industrial CO 2 feeds differ from most reported experiments. Although our main conclusions are likely transferable, the scale of recycle streams and separation units for a dilute CO 2 feed could change the optimum between separations and reactions. Lastly, to clarify reports of high SPC, we recommend reporting FE CO2R and SPC at the same conditions, rather than the best-case scenarios for each. It has been repeatedly shown that selectivity and SPC trade off in current MEA designs [23] , [29] . A singlestar plot should not include the best performance of an electrolyzer under multiple operating conditions. Given the (bi)carbonate equilibrium, we also note that conversions should always be reported as the ratio of CO 2 in CO 2 R products/CO 2 fed, and never CO 2 consumed/CO 2 fed. In summary, we analyzed stream compositions for state-of-the-art CO 2 electrolyzers to show that single-pass conversion alone does not capture the extent of downstream gas separations required. Although electrolyzers with high SPC do not dilute products in unreacted CO 2 , they still produce mixed cathode product streams. In current electrolyzer designs, this tradeoff arises from physical limitations. Low CO 2 feed flow rates and proton-rich environments maximize SPC but increase the side reaction of hydrogen evolution. We recommend that researchers prioritize and report outlet gas compositions, since maximizing product yield and mole fraction in the cathode outlet is more practically important than maximizing single-pass conversion. While reactor designs that decouple the tradeoff between selectivity and SPC could be pursued, electrolyzer energy dominates separation for both low and high SPC operation, so this is not the most pressing challenge facing CO 2 R scaleup. Thermocatalytic processes and solid oxide electrolytic cells often operate at low SPC with separation and recycle schemes, optimizing systems for the reaction rather than separation. CO 2 electrolyzers can similarly benefit from prioritizing other goals, including high product yields and low cell voltages, over increased single-pass conversion.